ATG5 defines a phagophore domain connected to the endoplasmic reticulum during autophagosome formation in plants Autophagosomes are the organelles responsible for macroautophagy and arise, in yeast and animals, from the sealing of a cup-shaped double-membrane precursor, the phagophore. How the phagophore is generated and grows into a sealed autophagosome is still not clear in detail, and unknown in plants. This is due, in part, to the scarcity of structurally informative, real-time imaging data of the required protein machinery at the phagophore formation site. Here we find that in intact living Arabidopsis tissue, autophagy-related protein ATG5, which is essential for autophagosome formation, is present at the phagophore site from early, sub-resolution stages and later defines a torus-shaped structure on a flat cisternal early phagophore. Movement and expansion of this structure are accompanied by the underlying endoplasmic reticulum, suggesting tight connections between the two compartments. Detailed real-time and 3D imaging of the growing phagophore are leveraged to propose a model for autophagosome formation in plants. Understanding compartment formation represents a fundamental challenge in cell biology. Macroautophagy (autophagy hereafter) is the delivery of cytosolic cargos entrapped by double-membrane bound vesicles, the autophagosomes, to lytic compartment(s) for bulk degradation. Present at all times at low levels, autophagosome formation is stimulated, among other instances, in the acute response to nutrient starvation, to allow reattribution of cellular resources [1] . Additional important roles for autophagy have been recently reviewed [2] , [3] . The importance of autophagy in physiology and development, and the unusual architecture of the autophagosome, have stimulated intensive research on the biogenesis of this compartment in yeast and mammals [4] , [5] . Many homologues of the ~30 genes required for autophagy in Saccharomyces cerevisiae —the Atg genes—are present in animals and plants. The recognition of the functional interactions among ATG proteins, and of the genetic requirements for their correct localization, has led to the proposal of a hierarchical order of action for the ATG proteins in yeast [6] and mammals [7] . In parallel, significant advance has also been made on the imaging of structures associated with autophagosome formation and delivery. Present challenges include full integration of molecular scaffolding data with in vivo localization and morphologically informative visualization of early autophagosomal structures in real-time and three dimensions [4] , [5] . Three major phases in the genesis of the autophagosome can be distinguished: nucleation, expansion and closure of a cisternal precursor, the phagophore. In the nucleation step, activity of the ATG1 protein kinase complex at the site of autophagosome formation allows for the enrichment of local membranes in phosphatidylinositol 3-phosphate (PtdIns(3)P) by phosphatidylinositol 3-kinase. In mammalian cells, these membranes, named omegasomes, are thought to represent either the precursor or an assembly platform for the phagophore [8] . PtdIns(3)P-enriched membranes are in turn required for the recruitment of ATG12-ATG5-ATG16 complexes, and these allow conjugation of ATG8 to phosphatidylethanolamine lipids present in the membrane of the phagophore [9] , [10] , [11] , [12] . Anchoring of ATG8 to the phagophore mediated by the ATG5-containing complex is thought to be required for membrane expansion and subsequent sealing of the phagophore [13] , [14] , [15] , [16] . Coherently, atg5 loss-of-function mutants are unable to form autophagosomes [17] , [18] . Although ATG8 is found on the autophagosome from its formation to its lytic destruction, the ATG5 complex has been shown to transiently label autophagosomal structures in yeast [19] , [20] and mammals [21] , [22] , leaving the autophagosomal membrane before its fusion with the lytic compartment. As the ATG5 complex should define the exact site of ATG8 insertion in the membrane of the forming autophagosome [23] , imaging ATG5 dynamics at high resolution and in real time can be expected to shed light on the spatial organization of early structures and on the cellular site of autophagosome formation. In yeast, autophagosomes are formed in close proximity of the vacuolar membrane, whereas in mammals early autophagosomal structures are connected with the endoplasmic reticulum (ER) [24] , [25] and with ER–mitochondria contact sites in particular [26] , [27] . However, interactions with the plasma membrane have also been reported [28] . Sites of autophagosome formation, and possibly membrane sources, could therefore vary in different physiological conditions and cell types [5] . In plants, autophagy has important roles in stress tolerance, senescence and grain filling [29] , [30] . The induction and conjugation machineries leading to ATG8 lipidation have been characterized [3] , [31] and autophagosomal structures identified employing fluorescence-tagged ATG8 (refs 13 , 29 ), ATG1 and ATG13 (ref. 32 ), the selective adaptor NBR1 (ref. 33 ), or the BAR-domain protein SH3P2 (ref. 34 ). However, despite other remarkable advances [35] , [36] , [37] , [38] , the different steps of the autophagic pathway are not resolved. Moreover, little information is presently available on the morphology of early autophagosomal structures [34] , and the subcellular distribution of the ATG5 complex or the site of autophagosome formation are currently unknown. To address these questions, we focused on ATG5 dynamics in differentiating root epidermal cells of Arabidopsis plants. These cells are characterized by a large central vacuole delimiting the cytosol to a 1- to 2-μm-thick cortical region below the plasma membrane and, as all epidermal cells in the root of Arabidopsis seedlings, can be readily subjected to live cell imaging and pharmacological treatments in the intact organ. Real-time and three-dimensional (3D) imaging of a biologically functional ATG5 fluorescent reporter in transgenic plants, in conjunction with ATG8 or ER reporters, allows us to identify unambiguously early autophagosomal structures (phagophores). We show that ATG5 defines a toroidal domain on the expanding phagophore, which appears as tightly connected to the outer face of the cortical ER network, facing the plasma membrane. Our observations can be integrated in a model for autophagosome formation, in which the ATG5 complex decorates the high curvature domain of the phagophore at all stages of its differentiation. In this model, ATG5 leaves the phagophore as its aperture is sealed and the neo-formed autophagosome simultaneously detaches itself from the ER. Autophagic induction of an ATG5-GFP subcellular pattern When autophagy was induced by nutrient starvation, the pattern of an ATG5-GFP reporter reorganized from a mainly diffused cytosolic signal, to a highly punctate one, including ring-like structures. In parallel, ATG8-labelled particles increased ( Fig. 1a–d ). Both changes were abolished by the PtdIns(3)-kinase inhibitor wortmannin, which impedes autophagosome formation [39] ( Fig. 1e,f ). We then tested whether ATG5 reporters were transported to the vacuole with the autophagosome, by applying the vacuolar ATPase inhibitor concanamycin A, which allows the accumulation of undegraded autophagic structures (autophagic bodies) by inactivating vacuolar proteases [13] . In contrast with the accumulation of ATG8-labelled autophagic bodies, no ATG5 signal was ever detected in the vacuole ( Fig. 1g,h ). Identical results were obtained employing mCherry-ATG8 ( Supplementary Fig. 1 ). Therefore, the observed ATG5 structures are induced similarly to ATG8-labelled autophagosomes, but do not follow these compartments until the vacuole. 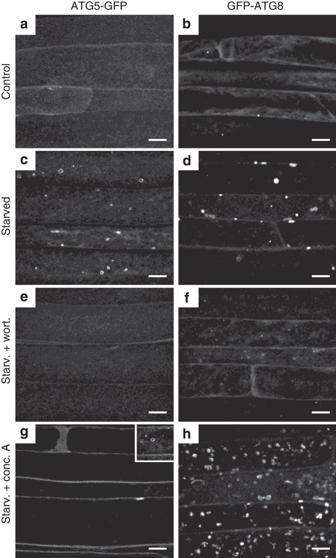Figure 1: Autophagic induction of the ATG5-GFP subcellular pattern. Confocal images of the GFP fluorescent patterns in seedlings expressing ATG5-GFP or GFP-ATG8. (a,b) Control conditions: cytosolic signal associated with rare fluorescent puncta. (c,d) High increase of fluorescent puncta after 2 h of nutrient starvation. Note ring-like ATG5 structures inc. (e,f) Wortmannin treatment blocks the occurrence of fluorescent ATG5 or ATG8 structures. (g,h) Maximum intensity projections of vacuolar focal planes, allowing visualization of autophagic bodies after 4 h of nutrient starvation in the presence of concanamycin A. Vacuolar ATG5-GFP fluorescence is not detected (g), while GFP-ATG8 signals are abundant (h). An inset ing, corresponding to a cortical focal plane, shows that formation of cytosolic ATG5 structures in the cytosol is not inhibited by concanamycin A treatment. Maximum intensity projections of 10-μm-deep deconvolved stacks, of cortical (a–f, and inset ing) or vacuolar focal planes (g,h). Scale bar, 10 μm. Figure 1: Autophagic induction of the ATG5-GFP subcellular pattern. Confocal images of the GFP fluorescent patterns in seedlings expressing ATG5-GFP or GFP-ATG8. ( a , b ) Control conditions: cytosolic signal associated with rare fluorescent puncta. ( c , d ) High increase of fluorescent puncta after 2 h of nutrient starvation. Note ring-like ATG5 structures in c . ( e , f ) Wortmannin treatment blocks the occurrence of fluorescent ATG5 or ATG8 structures. ( g , h ) Maximum intensity projections of vacuolar focal planes, allowing visualization of autophagic bodies after 4 h of nutrient starvation in the presence of concanamycin A. Vacuolar ATG5-GFP fluorescence is not detected ( g ), while GFP-ATG8 signals are abundant ( h ). An inset in g , corresponding to a cortical focal plane, shows that formation of cytosolic ATG5 structures in the cytosol is not inhibited by concanamycin A treatment. Maximum intensity projections of 10-μm-deep deconvolved stacks, of cortical ( a – f , and inset in g ) or vacuolar focal planes ( g , h ). Scale bar, 10 μm. Full size image Expression of the ATG5-GFP fusion in the atg5 mutant restored autophagic flux, as seen through the accumulation of vacuolar autophagic bodies in response to concanamycine A ( Fig. 2a ). This demonstrates that the ATG5 reporter is, at least in part, biologically functional, as also strongly suggested by the observation of identical fluorescence patterns in atg5 and wild-type plants, including characteristic ring-like structures ( Fig. 2b ). Immunoblotting indicates that the ATG5-GFP reporter is not overexpressed, and that it can be conjugated to ATG12, albeit to a lesser extent than the endogenous protein ( Supplementary Fig. 2 ). 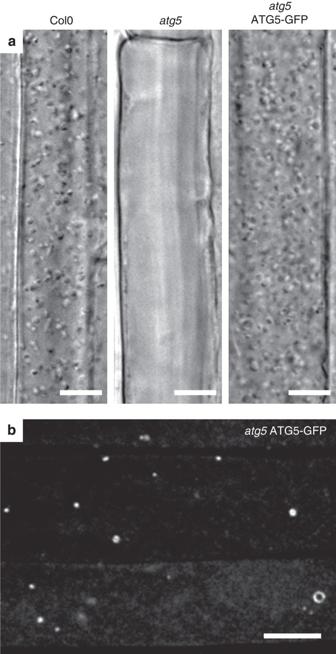Figure 2: Functional complementation of theatg5mutant by the ATG5-GFP reporter. (a) Differential interference contrast micrographs of root epidermal cells incubated for 8 h with concanamycin A, in nutrient starvation conditions. Autophagic bodies accumulation in the vacuole is clearly visible in wild-type seedlings, absent in theatg5-1mutant and restored inatg5-1seedlings expressing ATG5-GFP. (b) Confocal microscopy. The ATG5-GFP fluorescence pattern in theatg5-1background is identical to that observed in wild-type seedling, including ring-like structures. Scale bar, 15 μm. Figure 2: Functional complementation of the atg5 mutant by the ATG5-GFP reporter. ( a ) Differential interference contrast micrographs of root epidermal cells incubated for 8 h with concanamycin A, in nutrient starvation conditions. Autophagic bodies accumulation in the vacuole is clearly visible in wild-type seedlings, absent in the atg5-1 mutant and restored in atg5-1 seedlings expressing ATG5-GFP. ( b ) Confocal microscopy. The ATG5-GFP fluorescence pattern in the atg5-1 background is identical to that observed in wild-type seedling, including ring-like structures. Scale bar, 15 μm. Full size image An ATG5 ring identifies growing autophagosomal structures Interestingly, exception made for the smaller structures close in size to the optical resolution limit, ATG5-GFP appeared to always label a subdomain of the ATG8 particle ( Fig. 3a ). Different shapes were observed, including ATG5 ring-like structures. This partial overlap between ATG5 and ATG8 signals was never disrupted despite the dynamic context ( Supplementary Movie 1 ), suggesting that the two proteins label the same membrane, or distinct but tightly connected structures. Under nutrient starvation, 79% of ATG8-labelled structures were associated with an ATG5 signal, and, reciprocally, 95% of ATG5 signals partially overlapped ATG8 fluorescence in double transgenic ATG5-GFP mCh-ATG8 plants (see Supplementary Fig. 3 for additional quantifications). 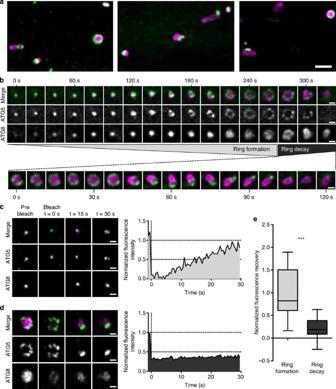Figure 3: An ATG5-labelled domain defines the growing phase of autophagosomal structures. (a) Dual observation of ATG5-GFP and mCh-ATG8 under nutrient starvation reveals a partial colocalization of the two reporters. Merge of the GFP (green) and ATG8 (magenta) channels of maximum intensity projections of 20-μm-deep deconvolved stacks. Scale bar, 3 μm. (b) Real-time imaging of an individual autophagosomal structure, showing one deconvolved image per 20 s. The ATG5 ring formation phase is defined as the steps up to establishment of the maximum diameter of the ring structure. The following steps, defined as the decay phase, being more dynamic, are depicted also at higher time resolution. Single-plane merged images of ATG5-GFP (green) and mCh-ATG8 (magenta) channels, deconvolved. Scale bar, 1 μm. (c) Representative FRAP experiment on mCh-ATG8 during the ring formation phase. Deconvolved images. Scale bar, 1 μm. The corresponding fluorescence recovery kinetic, measured on non-deconvolved images, is shown on the right. (d) Representative FRAP experiment of mCh-ATG8 during the ring decay phase, presented as inc. (e) Box and whiskers representations of fluorescence recoveries during ATG5 ring formation (n=11) and decay (n=17). Whiskers comprise the 10–90 percentile, the box the two central quartiles. The mean recovery values are indicated by an horizontal line. Recoveries during ATG5 ring formation and ring decay were significantly different according to the Mann–Whitney statistical test (***P<0.001). Figure 3: An ATG5-labelled domain defines the growing phase of autophagosomal structures. ( a ) Dual observation of ATG5-GFP and mCh-ATG8 under nutrient starvation reveals a partial colocalization of the two reporters. Merge of the GFP (green) and ATG8 (magenta) channels of maximum intensity projections of 20-μm-deep deconvolved stacks. Scale bar, 3 μm. ( b ) Real-time imaging of an individual autophagosomal structure, showing one deconvolved image per 20 s. The ATG5 ring formation phase is defined as the steps up to establishment of the maximum diameter of the ring structure. The following steps, defined as the decay phase, being more dynamic, are depicted also at higher time resolution. Single-plane merged images of ATG5-GFP (green) and mCh-ATG8 (magenta) channels, deconvolved. Scale bar, 1 μm. ( c ) Representative FRAP experiment on mCh-ATG8 during the ring formation phase. Deconvolved images. Scale bar, 1 μm. The corresponding fluorescence recovery kinetic, measured on non-deconvolved images, is shown on the right. ( d ) Representative FRAP experiment of mCh-ATG8 during the ring decay phase, presented as in c . ( e ) Box and whiskers representations of fluorescence recoveries during ATG5 ring formation ( n =11) and decay ( n =17). Whiskers comprise the 10–90 percentile, the box the two central quartiles. The mean recovery values are indicated by an horizontal line. Recoveries during ATG5 ring formation and ring decay were significantly different according to the Mann–Whitney statistical test (*** P <0.001). Full size image Time-lapse acquisitions of individual growing autophagosomal structures ( n =70) revealed one similar sequence of events ( Fig. 3b ). Isolated ATG5 puncta (<0.3 μm) recruited an ATG8 signal and drastically increased in size, evolving distinct patterns for the two reporters. The ATG5 signal systematically formed a growing ring surrounding an ATG8-labelled region, finally reaching a diameter of up to 2 μm. We termed these steps of autophagosome formation ‘the ring formation phase’. Strikingly, ATG5 ring-like structures appeared systematically in a plane parallel to the cell surface (either the apical or the lateral one) and were rather static on the vertical axis within the cell, suggesting the existence of physical constraints for their positioning. In the subsequent, shorter, ‘ring decay phase’, the ATG5 domain appeared to rapidly collapse, as the whole structure tended to become more mobile to finally disappear from the focal plane, presumably by rapidly fusing with the vacuole, as if detached from an anchor (also see Supplementary Movies 2–4 ). Fluorescence recovery after photobleaching (FRAP) experiments on mCh-ATG8 demonstrated a net recruitment of mCh-ATG8 on the autophagosomal structure during the ring formation phase ( Fig. 3c ). The slow recovery kinetics reflects, as expected, a process not uniquely based on diffusion from the cytosol. In the ring formation phase, in several cases recovery exceeded 100%, reflecting a growing structure. In contrast, recovery was weaker or even negative during the ring decay phase, indicating in this case the departure of ATG8 from the autophagosomal membrane ( Fig. 3d,e ). 3D reconstruction of the growing phagophore A faithful 3D representation of these evolving structures was obtained employing an imaging strategy compatible with both the dynamic nature of the autophagosome and the weak signal of the ATG5-GFP reporter. Representative objects generated by 3D surface rendering are presented in Fig. 4a , disposed along the temporal sequence defined by our real-time observations. The first structures giving rise to a discernible ATG5 ring in two-dimensional (2D) imaging were revealed in 3D as distinctly planar objects, in which the ATG8 signal was always surrounded by an expanding ATG5 torus (structure I in Fig. 4a,b ). Subsequently, further growth expands the object in the three dimensions, with the ATG5 reporter surrounding a region devoid of ATG8 signal (structure II in Fig. 4a,b ), suggesting that ATG5 is positioned at the aperture of the growing phagophore. These observations also demonstrate that ATG5 defines, in 3D, a toroidal domain of the phagophore. Such pattern is different from more commonly seen ring-like signals, which correspond to the optical section, or the z -projection, of hollow spherical objects. Finally, objects in late steps of the ATG5 ring decay phase reveal their higher mobility and deformation, and are peripherally labelled by the mCherry reporter, reflecting the expected anchoring of ATG8 to the autophagosomal membrane (structures III and IV in Fig. 4 ). 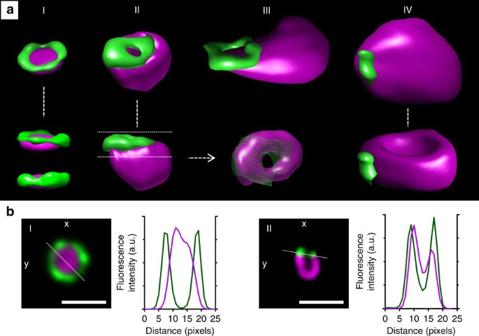Figure 4: Three-dimensional reconstructions of the growing phagophore. (a) Three-dimensional surface rendering of deconvolved stacks of ATG5 (green) and ATG8 (magenta) domains on the forming autophagosome. Four representative objects are shown, disposed left to right according to a temporal sequence deduced from integration of real-time data on individual structures. Additional views are presented below structures I, II and IV. Note the planarity of structure I, the first morphologically informative object in the ATG5 ring formation phase, evident in two profile views. In structure II, the ATG5 torus is disposed around the aperture of the phagophore, as clearly seen with a top view of the reconstruction of the upper third of the object (arrow, green mesh for the ATG5 surface). In structure IV, corresponding to a late step in the ATG5 ring decay phase, the cavity of the neo-formed autophagosome is detectable in the additional mid-section. (b) Two-dimensional horizontal views of representative structures of type I and II, corresponding to the planes of maximum ATG5 intensity of thez-stacks. Fluorescence intensity profiles along a line crossing the confocal image confirm the disposition of ATG5-GFP and mCh-ATG8 visible in the 3D surface reconstructions. Scale bar, 2 μm. Figure 4: Three-dimensional reconstructions of the growing phagophore. ( a ) Three-dimensional surface rendering of deconvolved stacks of ATG5 (green) and ATG8 (magenta) domains on the forming autophagosome. Four representative objects are shown, disposed left to right according to a temporal sequence deduced from integration of real-time data on individual structures. Additional views are presented below structures I, II and IV. Note the planarity of structure I, the first morphologically informative object in the ATG5 ring formation phase, evident in two profile views. In structure II, the ATG5 torus is disposed around the aperture of the phagophore, as clearly seen with a top view of the reconstruction of the upper third of the object (arrow, green mesh for the ATG5 surface). In structure IV, corresponding to a late step in the ATG5 ring decay phase, the cavity of the neo-formed autophagosome is detectable in the additional mid-section. ( b ) Two-dimensional horizontal views of representative structures of type I and II, corresponding to the planes of maximum ATG5 intensity of the z -stacks. Fluorescence intensity profiles along a line crossing the confocal image confirm the disposition of ATG5-GFP and mCh-ATG8 visible in the 3D surface reconstructions. Scale bar, 2 μm. Full size image A tight and asymmetrical connection to cortical ER Next, to investigate whether the ER cortical network might interact with the growing phagophore and provide the hypothesized anchoring platform, ATG5 and ATG8 reporters were co-imaged with the luminal ER marker GFP-HDEL [40] . ATG5-mCh or mCh-ATG8 and GFP-HDEL signals were systematically superposed, even in time-lapse acquisitions, suggesting an interaction with cortical ER, which appears as a highly dynamic network of tubular and cisternal domains ( Fig. 5a,f and Supplementary Movies 5–6 ). Remarkably, all ATG5-mCh signals, that is, smaller dot-like structures (corresponding either to early formation stages, or to late ring decay structures, as seen in Fig. 3b ), and the larger tori were detected close to the ER and almost exclusively on the outer face (that is, facing the plasma membrane) in the proximity of cisternal domains ( Fig. 5b–e ). Coherently, smaller ATG8-labelled structures, globally representing the earlier stages of autophagosome formation, were also positioned on the outer face of the ER, as for ATG5 ( Fig. 5i ). In contrast, most of the mCh-ATG8 structures were tightly embedded in the underlying ER sheets, which appeared to form a cradle accompanying the expanding phagophores ( Fig. 5g,h,j ). Such deformations of ER sheets accompanying growth of the larger autophagosomal structures were evident in 2D as high intensity GFP-HDEL ring-like sectional signals ( Fig. 5f ). Optical resolution is sufficient to exclude the systematic presence of GFP-HDEL in the autophagosome’s content. In agreement with this observation, GFP-HDEL signal was not detected in autophagic bodies accumulating in the vacuole ( Supplementary Fig. 4 ). 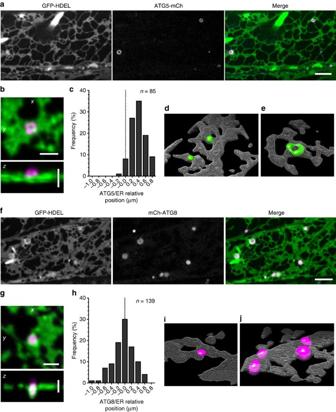Figure 5: Close association of the phagophore with the external face of cortical ER. (a) Single-plane images captured on a cortical plane in a GFP-HDEL ATG5-mCh stably transformed plant. ATG5 structures are systematically superposed with the ER luminal marker GFP-HDEL. Bright fusiform structures visible with the latter are ER bodies, typical ofBrassicacaeplants. SeeSupplementary Movie 5for a time lapse of a forming ATG5 torus. Scale bar, 5 μm. (b) Maximum intensity projections of a 5-μm-deep deconvolvedz-stack, on thex,yandx,zplanes, showing a typical ATG5 torus. Note how the ATG5 torus is placed on the upper/outer face of the ER with respect to the GFP-HDEL signal. Scale bar, 2 μm. (c) Frequency distribution of the difference in microscope stagez-positions between the maxima of fluorescence intensities for ATG5-mCh and GFP-HDEL. The maximum-intensityz-position of virtually all the ATG5 structures analysed is placed on the upper, outer face of the ER. (d) Three-dimensional surface rendering of early, dot-like ATG5-mCh structures (green), disposed on the ER cortical network (grey meshes). (e) An ATG5-mCh torus placed on the outer, upper face surface of the ER. (f) mCh-ATG8 signals are superposed with GFP-HDEL. Note how the ER luminal marker reveals structured ER domains at the positions of autophagosomal structures labelled by mCh-ATG8 (see alsoSupplementary Movie 6). Scale bar, 5 μm. (g) Maximum intensity projections of a 5-μm-deep deconvolvedz-stack, on thex,yandx,zplanes, showing a typical mCh-ATG8 labelled structure embedded in an ER cradle. Scale bar, 2 μm. (h) As inc, this time showing the relative positions of the maxima of mCh-ATG8 intensity along thezaxis relative to GFP-HDEL. ATG8 structures are more deeply embedded in the ER compared with ATG5. (i) Three-dimensional surface rendering of early, dot-like mCh-ATG8 structures (magenta) disposed on the outer, upper face of the ER cortical network (grey meshes) and (j) larger growing structures deeply embedded in the ER. Figure 5: Close association of the phagophore with the external face of cortical ER. ( a ) Single-plane images captured on a cortical plane in a GFP-HDEL ATG5-mCh stably transformed plant. ATG5 structures are systematically superposed with the ER luminal marker GFP-HDEL. Bright fusiform structures visible with the latter are ER bodies, typical of Brassicacae plants. See Supplementary Movie 5 for a time lapse of a forming ATG5 torus. Scale bar, 5 μm. ( b ) Maximum intensity projections of a 5-μm-deep deconvolved z -stack, on the x , y and x , z planes, showing a typical ATG5 torus. Note how the ATG5 torus is placed on the upper/outer face of the ER with respect to the GFP-HDEL signal. Scale bar, 2 μm. ( c ) Frequency distribution of the difference in microscope stage z -positions between the maxima of fluorescence intensities for ATG5-mCh and GFP-HDEL. The maximum-intensity z -position of virtually all the ATG5 structures analysed is placed on the upper, outer face of the ER. ( d ) Three-dimensional surface rendering of early, dot-like ATG5-mCh structures (green), disposed on the ER cortical network (grey meshes). ( e ) An ATG5-mCh torus placed on the outer, upper face surface of the ER. ( f ) mCh-ATG8 signals are superposed with GFP-HDEL. Note how the ER luminal marker reveals structured ER domains at the positions of autophagosomal structures labelled by mCh-ATG8 (see also Supplementary Movie 6 ). Scale bar, 5 μm. ( g ) Maximum intensity projections of a 5-μm-deep deconvolved z -stack, on the x , y and x , z planes, showing a typical mCh-ATG8 labelled structure embedded in an ER cradle. Scale bar, 2 μm. ( h ) As in c , this time showing the relative positions of the maxima of mCh-ATG8 intensity along the z axis relative to GFP-HDEL. ATG8 structures are more deeply embedded in the ER compared with ATG5. ( i ) Three-dimensional surface rendering of early, dot-like mCh-ATG8 structures (magenta) disposed on the outer, upper face of the ER cortical network (grey meshes) and ( j ) larger growing structures deeply embedded in the ER. Full size image Autophagosomal structures were also visualized by transmission electron microscopy, employing different sample preparation methods, correlative light-electron microscopy and immunolabelling ( Fig. 6 ). All approaches revealed close contacts of autophagosomal structures with ER-like membranes, further indicating an important role of the ER in autophagosome formation. 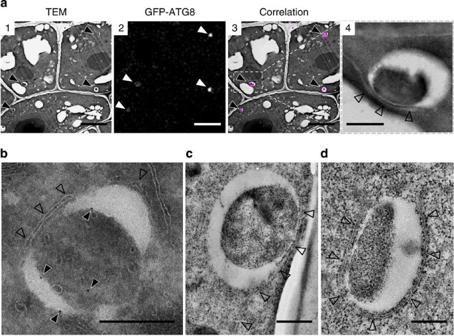Figure 6: Close contacts between autophagosomes and ER membranes. (a) Correlative light-electron microscopy of GFP-ATG8-labelled autophagosomal structures. Correlation of a TEM micrograph of a root transverse section (1) with fluorescent imaging of GFP-ATG8 (arrowheads, 2) confirms the association of ATG8 signal with autophagosome (3). A closer view shows close contacts with ER-like membranes (empty arrowheads, 4). (b) Immunogold labelling of GFP-ATG8 on cryosections, employing an anti-GFP antibody (arrowheads). Similar interactions between ER membranes and autophagosomal structures can be detected either on cryofixed (samples c) or after chemical fixation (d). Empty arrowheads: connections with ER-like membranes. Scale bars, 5 μm ina(1–3); 0.5 μm ina(4) andb(1–3). Figure 6: Close contacts between autophagosomes and ER membranes. ( a ) Correlative light-electron microscopy of GFP-ATG8-labelled autophagosomal structures. Correlation of a TEM micrograph of a root transverse section (1) with fluorescent imaging of GFP-ATG8 (arrowheads, 2) confirms the association of ATG8 signal with autophagosome (3). A closer view shows close contacts with ER-like membranes (empty arrowheads, 4). ( b ) Immunogold labelling of GFP-ATG8 on cryosections, employing an anti-GFP antibody (arrowheads). Similar interactions between ER membranes and autophagosomal structures can be detected either on cryofixed (samples c) or after chemical fixation ( d ). Empty arrowheads: connections with ER-like membranes. Scale bars, 5 μm in a (1–3); 0.5 μm in a (4) and b (1–3). Full size image The toroidal disposition of ATG5 defining the growing edges of the plant phagophore has not been reported in other organisms. In mammalian cells and yeast, ATG5 was mainly found homogenously distributed onto early phagophores, shifting to a preferential localization on the whole outer surface of maturing phagophores [7] , [21] , [22] . However, a recent study in yeast describes a dot-like localization of Atg5 juxtaposed to the Atg8 signal [41] , which is consistent with our observation of a fine regulation of the spatial disposition of ATG5 on the phagophore/isolation membrane. Although our findings could reflect plant-specific aspects of phagophore formation, the possibility that the toroidal disposition of ATG5 has not been detected yet in other models for technical reasons cannot be formally excluded. It will be interesting to establish whether interactions with ATG12, or other molecular partners, are required for the observed localization of ATG5. In this respect, we noticed that only a fraction of the ATG5-GFP reporter appears to be conjugated to ATG12. However, small amounts of Atg12-Atg5-GFP conjugate could very well generate a detectable signal once concentrated on the phagophore. When considering the kinetics of the establishement of ATG5 structures, the appearance of the ATG5 torus as the enlargement of sub-resolution puncta indicates recruitment of ATG5 at a very early stage of the plant autophagic pathway. Such behaviour is also suggested by recent temporal analysis in mammalian cells, showing co-recruitment of ATG5 with ATG1/ULK1 at the phagophore initiation site [22] . Interestingly, the mammalian PtdIns(3)P-enriched omegasome membranes were also visualized as ring-like structures positioned close to, but not overlapping with, ATG5 signals, employing the PtdIns(3)P-binding protein DFCP1. However, no data describing positioning of the DFCP1 ring relative to phagophore aperture were obtained [8] . A tight physical connection of the ATG5 torus to peripheral ER is suggested by our time-lapse observations. The polarity of this interaction, with systematic positioning of the ATG5 torus on the external face of the ER, was unexpected. This might reflect either intrinsic polarity of ER domains involved and/or further interactions with other cell components, for example, the cortical microtubule network or the plasma membrane. Our experiments did not directly address the question of whether the observed ATG5 torus is positioned directly on peripheral ER or on a neighbouring membrane. However, the localization of ATG5 on the edge of a flat membranous cisterna, growing because of lipid deposition or synthesis, could explain the observed geometric regularity of the expanding ATG5 pattern. The maintenance of a flat early phagophore structure would be imposed by anchoring to underlying ER, which could possibly also act as a lipid provider. The observed cup-like deformation of the ER cisternae underlying, at later stages, the expanding phagophore are consistent with this view, and also imply physical connections resisting the forces exerted by the growing phagophore. Finally, it will be interesting to establish whether, as suggested by our time-course observations, shrinkage and collapse of the ATG5 domain are concomitant with sealing of the autophagosome and its departure from the ER. Indeed, as the yeast ATG5 complex has membrane tethering capabilities [11] , it is tempting to speculate that such complex could also be involved in tethering the phagophore membrane to the underlying ER membrane, and in controlling sealing of the phagophore aperture. The idea of an additional role for ATG5 complexes, beside catalysis of ATG8 lipidation, is consistent with recent work showing that ATG12-ATG5-ATG16 complexes and lipidated ATG8 can assemble in a functionally relevant 2D meshwork on membranes [42] . It is therefore possible that regulated formation and disassembly of such meshwork at the ATG5-labelled domain of the phagophore underlie the control of its expansion and closure, in interaction with the cargo. It will be important to characterize the domain labelled by ATG5 at the electron microscopy level, albeit this represents a difficult technical challenge, as ATG5 labels a small fraction of the phagophore. Our electron microscopy observations ( Fig. 6 ) reinforce the concept of a tight interaction of the phagophore with the underlying ER membranes, an interaction that has also been recently suggested with the localization of the SH3P2 protein on autophagosome-related structures by immunoelectron microscopy [34] . Interactions between omegasomes, isolation membranes and the ER are well documented in mammalian cells [8] , [24] , [25] , [43] . Notably, the continuity of the isolation membrane with the ER led to a model implying direct differentiation of the phagophore from this compartment, and the systematic inclusion of ER fragments in the autophagosome, captured by folding and invagination of the isolation membrane, sandwiched between cradle-shaped ER sheets [25] . However, the mammalian isolation membrane–ER cradle model for autophagosome formation may not be transposable to plants, as systematic inclusion of ER fragments was not observed in this work. We propose that during macroautophagy in plants, the ATG5 complex decorates the high-curvature edge of a cisternal-like early phagophore anchored to the ER ( Fig. 7 ). The asymmetric nature of the interaction of the phagophore with the ER would in turn provide the initial polarity required for establishment of the membrane curvature of the growing phagophore. How the initial planar, cisternal-like phagophore is established, grows into a cup-like structure and how ATG5 is removed from the phagophore at the end of its expansion are additional open questions deserving further investigation. 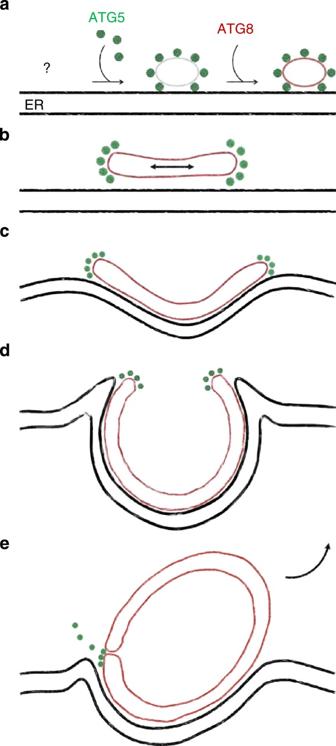Figure 7: Model of autophagosome formation during plant macroautophagy. (a) The growing phagophore, first detected as an ATG5-labelled (green) sub-resolution structure on the external surface of the ER, could directly differentiate from the ER, or derive from vesicular transport and fusion events. (b) After rapidly recruiting ATG8 (magenta), the initial phagophore expands as a mostly planar cisterna, whose toroidal edge is decorated by the ATG5 complex. It is not known whether a membrane continuum with the ER exists at this stage. ATG5, ATG8 and the ER co-evolve dynamically as if physically connected. (c,d) As the phagophore cisterna becomes cup-shaped and expands in the three dimensions, an accompanying ER cradle is formed. The ATG5 torus now encircles the phagophore’s aperture. (e) Finally, three events, which appear to take place simultaneously, might be mechanistically connected: ATG5 leaves the structure, the phagophore membrane is sealed and the neo-formed autophagosomes leaves the ER. Note that in this model ATG5 is always placed on membrane domains characterized by a high positive curvature, and how absence of ATG5 from the lumen of the sealed autophagosome is a logical consequence of this property. The asymmetric nature of the interaction of the phagophore with the ER could also explain the asymmetric fates observed for the inner and outer membranes of the autophagosome. Figure 7: Model of autophagosome formation during plant macroautophagy. ( a ) The growing phagophore, first detected as an ATG5-labelled (green) sub-resolution structure on the external surface of the ER, could directly differentiate from the ER, or derive from vesicular transport and fusion events. ( b ) After rapidly recruiting ATG8 (magenta), the initial phagophore expands as a mostly planar cisterna, whose toroidal edge is decorated by the ATG5 complex. It is not known whether a membrane continuum with the ER exists at this stage. ATG5, ATG8 and the ER co-evolve dynamically as if physically connected. ( c , d ) As the phagophore cisterna becomes cup-shaped and expands in the three dimensions, an accompanying ER cradle is formed. The ATG5 torus now encircles the phagophore’s aperture. ( e ) Finally, three events, which appear to take place simultaneously, might be mechanistically connected: ATG5 leaves the structure, the phagophore membrane is sealed and the neo-formed autophagosomes leaves the ER. Note that in this model ATG5 is always placed on membrane domains characterized by a high positive curvature, and how absence of ATG5 from the lumen of the sealed autophagosome is a logical consequence of this property. The asymmetric nature of the interaction of the phagophore with the ER could also explain the asymmetric fates observed for the inner and outer membranes of the autophagosome. Full size image DNA constructs To generate translational fusions of Arabidopsis ATG5 with green fluorescent protein (GFP) and mCherry, the coding region of ATG5 (gene AT5G17290 ) was amplified by PCR (primers 5′-TACAAAAAAGCAGGCTTCATGGCGAAGGAAGCGGTCAAG-3′ and 5′-CAAGAAAGCTGGGTCCCTTTGAGGAGCTTTCACAAG-3′), from a full-length complementary DNA provided by Dr K.Yoshimoto (IJPB, INRA Versailles, France) and introduced in pDONOR207 by Gateway BP reaction (Invitrogen). A pDONOR207 vector carrying the complete coding sequence of Arabidopsis ATG8e (gene AT2G45170 ) was provided by Dr C. Masclaux-Daubresse (IJPB, INRA Versailles). The ATG5 and ATG8e inserts of pDONOR207 were verified by sequencing and transferred by LR Recombinase reactions to binary vectors pMDC83 and pMDC43 (ref. 44 ) to generate ATG5-GFP and GFP-ATG8 fusions, transcribed by the 35S promoter. ATG5-mCh and mCh-ATG8 fusions were obtained through similar reactions with modified versions of pMDC83 and pMDC43 carrying the mCherry coding region in place of GFP, provided by Dr Sylvain Merlot (ISV,CNRS Gif-sur-Yvette, France). All constructs were verified by sequencing. Arabidopsis lines To generate Arabidopsis lines stably expressing ATG5-GFP, ATG5-mCh, GFP-ATG8 and mCh-ATG8 translational fusions, plants of the Columbia ecotype were transformed by the floral dip method [45] employing AGL0 Agrobacterium tumefaciens strains carrying the relevant plasmid. Single insertion homozygous families were selected by scoring for hygromycin resistance and fluorescence of the reporter protein. Plants stably expressing ATG5-GFP in the atg5-1 mutant [17] (SAIL_129_B07) for complementation experiments were generated by crossing and selecting the double homozygous F3 families by hygromycin resistance and PCR genotyping. Lines stably expressing both ATG5-GFP and mCh-ATG8 were generated by crossing and selecting the double homozygous F3 families by PCR genotyping and fluorescence of the reporter. Plants stably expressing GFP-HDEL (Arabidopsis Biological Resource Centre CS16251, corresponding to ER-gk [40] ) were crossed with the ATG5-mCh or the mCh-ATG8e lines to obtain the corresponding double-labelled plants. F1 seedlings issued from these crosses were directly employed. Growth conditions, autophagy induction and chemical treatments Seeds were surface sterilized in 70% (v/v) ethanol, 0.05% (v/v) Tween-20 for 10 min and stratified on growth medium for 2 days at 4 °C in the dark. Growth medium: half strength Murashige and Skoog solid medium composed of 2.15 g l −1 MS Basal Salt Mixture (Sigma, M5524); 1% (w/v) sucrose; 3 mM 2-(N-morpholino)ethanesulphonic acid, pH 5.6 and 3 g l −1 Gelzan (Sigma, G1910). Seedlings were grown vertically for 5 days in plates sealed with gas-permeable medical tape (Urgo Medical) in a growth chamber at 22 °C with a 16-h light/8-h dark photoperiod (300 μE m 2 s -1 ) and 65% relative humidity. To induce autophagy, 5-day-old seedlings were transferred to Petri dishes containing a 2.5-mm thin layer of half strength Murashige and Skoog liquid medium, depleted for nitrogen and carbon: Murashige and Skoog micronutrient salts (Sigma, M0529), 3 mM CaCl 2 , 1.5 MgSO 4 , 5 mM KCl, 1.25 mM KH 2 PO 4 , 0.5% (w/v) mannitol, 3 mM 2-(N-morpholino)ethanesulphonic acid, pH 5.6, for 2 h in the dark, with gentle rotatory shaking at 100 r.p.m. (nutrient starvation conditions). Controls were incubated similarly, employing normal half-strength MS liquid medium and in the light. For concanamycin A (Fluka, 27689) and wortmannin (Sigma, W1628) treatments, liquid medium was supplemented with, respectively, 1 and 30 μM of the chemical, diluted from frozen aliquoted stocks in dimethyl sulphoxide. Concanamycin A was added for the whole duration of the starvation treatment, while wortmannin was added only for the last 1 h. An equivalent volume of dimethyl sulphoxide was added to the controls. Immunoblotting Proteins were extracted from 7-day-old in vitro grown seedlings, after 2 h of nutrient starvation, or after incubation in nutrient-rich media, as indicated. Equal amounts, in fresh weight, of dissected roots were frozen in liquid nitrogen, disrupted with stainless steel beads (TissueLyser, Qiagen) and homogenized in extraction buffer, at a ratio of 5 μl mg −1 fresh weight. Extraction buffer was composed of 60 mM Tris-Cl pH 7.5, 10% (v/v) glycerol, 2% SDS, 2 mM phenylmethyl sulphonyl fluoride and 10 mM iodoacetamide. After migration on 10% SDS–PAGE and transfer to nitrocellulose (Amersham Hybond-C extra, GE Healthcare), membranes were treated with anti-ATG5 rabbit serum [17] at 1:4,000 dilution, or with an anti-GFP mouse monoclonal (JL-8, Invitrogen) at 1:2,000 dilution, using standard methods. As a control, anti-TSN serum [46] was employed at 1:4,000 dilution. Peroxidase activity coupled to the goat anti-rabbit secondary antibody (Calbiochem; 1:20,000 dilution) or rabbit anti-mouse secondary antibody (Calbiochem; 1:10,000 dilution) was revealed with an enhanced chemiluminescence kit (Millipore) following the manufacturer’s instructions. In the immunoblot processed with anti-ATG5 serum shown in Supplementary Fig. 2b , the membrane was directly imaged. Light microscopy All observations were done on root epidermal cells of the early differentiation zone, employing 5-day-old seedlings mounted in culture medium. To avoid unwanted autophagy induction, observation time under the microscope never exceeded 15 min after the plants were mounted. Confocal images were acquired with a Nipkow Spinning Disk confocal system (Yokogawa CSU-X1-A1) mounted on a Nikon Eclipse Ti E inverted microscope, equipped with a × 60 Apochromat TIRF oil-immersion objective (numerical aperture (NA): 1.49) and a × 100 Apochromat TIRF oil-immersion objective (NA: 1.49). Blue (491 nm Cobolt Calypso DPSS, 100 mW) and Yellow (561 nm Cobolt Jive DPSS, 150 mW) lasers were used for excitation of GFP and mCherry, respectively. A dual-band dichroic mirror (491/561 nm, Chroma) was used and band-pass filters of 525/45 nm and 607/36 nm (Semrock) allowed the detection of GFP and mCherry, respectively. Images were recorded with a EMCCD Evolve camera (Photometrics). The whole system was driven by MetaMorph software version 7.7 (Molecular Devices). For the simultaneous observation of GFP and mCherry, we employed a Dual View DV2 emission splitting device (Photometrics), equipped with a spectral module (Chroma) composed of a dichroic mirror 565 nm and band-pass filters for GFP (ET525/50m) and mCherry (ET630/75m). For 3D imaging, stacks were acquired with a z -step of 200 nm. Differential interferential contrast acquisitions were collected on a Leica SP8X equipped with an HC PL Apochromat × 63 oil-immersion objective (NA: 1.40). Image processing and analysis Image manipulation (cropping, projections, bleaching correction in time series), intensity measurements and particle counts were done with ImageJ (Wayne Rasband, National Institutes of Health). Fluorescent structures counts presented in Supplementary Fig. 3 were obtained manually, on maximum intensity projections of 15-μm-deep stacks, acquired on 7 seedlings for each condition. When indicated, images were deconvolved employing the Huygens Essential package (Scientific Volume Imaging, Hilversum, The Netherlands), with the following parameters: algorithm, CMLE; signal/noise ratio,10; quality threshold, 0.01%; maximum iterations, 100; background calculation, in/near objects. Three-dimensional surface rendering of deconvolved z -stacks was performed with the UCSF Chimera software [47] version 1.8 (Resource for Biocomputing, Visualization and Informatics at the University of California, San Francisco, supported by NIGMS P41-GM103311). Statistical analysis was executed with Prism software version 5.0 (GraphPad). The P -value is indicated as following: * P <0.05; ** P <0.01; *** P <0.001. FRAP analysis FRAP experiments were performed employing the ‘FRAP on the fly’ mode of an iLAS [2] module (Roper Scientifics). mCherry was selectively photobleached and structures were followed in time and space by keeping the GFP signal in focus, employing the DV2 emission splitter. Analysis involved five steps as follows: (1) total intensity along the time series were normalized to the total intensity of the first slice to correct for long-term loss of fluorescence under normal observation; (2) intensity of the bleached region was quantified by manually placing a round region of interest on the GFP signal, at each time point; (3) background was measured in an annular region surrounding the central region of interest and subtracted; (4) corrected intensity values were normalized to the pre-bleach level, estimated as the median of the nine time points preceding the photobleaching; (5) fluorescence recovery at 30 s was measured by linear interpolation. Electron microscopy The apical 3 mm of 5-day-old roots were prepared for correlative light-electron microscopy by the Tokauyasu method [48] essentially as described [49] , with the following modifications: we employed 3% paraformaldehyde and 0.1% glutaraldehyde in cacodylate buffer (0.1 M, pH 6.8) and replaced polyvinylpyrrolidone with methylcellulose. Ultrathin (90 nm) sections (Ultracut UC6, Leica) were collected on formwar and carbon-coated nickel or copper grids. For immunolabelling, sections were treated with anti-GFP antibodies (ab290, Abcam; 1:50 dilution) and anti-rabbit 10 nm gold conjugate IgG (BBinternational, 1:50 dilution) following published procedures [49] . For correlative microscopy, the grids were placed on a glass slide, GFP signals were collected by confocal microscopy and samples were then post-stained by aqueous 2% uranyl acetate and lead citrate. For complementary ultrastructural studies, the roots were chemically fixed and embedded in LRWhite resin as described [50] . All samples were observed at 120 kV with a JEOL 1400 electron microscope. How to cite this article: Le Bars, R. et al. ATG5 defines a phagophore domain connected to the endoplasmic reticulum during autophagosome formation in plants. Nat. Commun. 5:4121 doi: 10.1038/ncomms5121 (2014).